PTEN regulates DNA replication progression and stalled fork recovery Faithful DNA replication is a cornerstone of genomic integrity. PTEN plays multiple roles in genome protection and tumour suppression. Here we report on the importance of PTEN in DNA replication. PTEN depletion leads to impairment of replication progression and stalled fork recovery, indicating an elevation of endogenous replication stress. Exogenous replication inhibition aggravates replication-originated DNA lesions without inducing S phase arrest in cells lacking PTEN, representing replication stress tolerance. iPOND analysis reveals the physical association of PTEN with DNA replication forks and PTEN-dependent recruitment of Rad51. PTEN deletion results in Rad51 dissociation from replication forks. Stalled replication forks in Pten -null cells can be reactivated by ectopic Rad51 or PTEN, the latter facilitating chromatin loading of Rad51. These data highlight the interplay of PTEN with Rad51 in promoting stalled fork restart. We propose that loss of PTEN may initiate a replication stress cascade that progressively deteriorates through the cell cycle. PTEN is crucial in tumour suppression, controlling a wide range of cellular signals and processes [1] . In addition to the canonical function of antagonizing the PI3K/AKT signalling pathway, increasing evidence points to the intriguing role of PTEN in genomic stability. PTEN maintains the structural integrity of chromosomes and regulates DNA damage repair [2] , [3] , [4] . In addition, our recent work reveals the interplay of PTEN with histones in chromatin remodelling [5] . PTEN is also a critical factor in cell cycle regulation and checkpoint control. For example, loss of PTEN promotes cell cycle progression from G0 to G1 [6] , while overexpression of PTEN induces G1 arrest [7] , [8] . PTEN -null cells exhibit G2 checkpoint defects in response to ionizing radiation due to CHK1 phosphorylation and dislocation [9] . These studies demonstrate that PTEN regulates G1 and G2 progression. During the cell cycle, DNA replication and chromosome segregation require meticulous control mechanisms to ensure genomic integrity. PTEN regulates mitotic proteins through the APC-CDH1-mediated cellular senescence pathway [10] . Recent reports suggest the involvement of PTEN in the regulation of centrosome maturation [11] and the mitotic checkpoint [12] . Faithful genetic transmission relies on DNA replication during S phase and segregation of sister chromatids during M phase. These two processes are intertwined such that errors found in one phase may originate from the other. Replication stress is defined as the slowing or stalling of replication fork progression and has emerged as a major source of genomic instability [13] . In addition to exogenous replication stress caused by replication blocking agents, replication stress can arise from endogenous sources such as the accumulation of metabolic byproducts or an increase in chromosomal fragility due to deficiency of the genome surveillance system. Replication stress may stall chromosome duplication, leaving chromosomal segments unreplicated when cells enter mitosis [14] . Unreplicated DNA often forms anaphase bridges that impede chromosome segregation and thereby challenge the stability of the whole genome. In this study, we find that loss of PTEN gives rise to increased frequencies of mitotic anaphase bridges resulting from DNA lesions generated during replication. Further investigation of replication fork behaviour reveals spontaneous defects of fork progression upon PTEN depletion. In response to exogenous replication perturbation, DNA fibres in PTEN -null cells fail to restart. These data demonstrate that PTEN is important in promoting elongation of newly synthesized DNA strands and plays an essential role in the recovery of stalled forks when replication is challenged by exogenous replication stress. PTEN -deficient cells exhibit defective DNA replication Our earlier studies have shown structural and numerical chromosomal instability in cells lacking functional PTEN [2] , [15] . In order to investigate chromosomal segregation errors during mitosis, we depleted PTEN in HeLa cells by short hairpin RNA (shRNA) ( Supplementary Fig. 1a ) and observed a significantly higher frequency of anaphase bridges and lagging chromosomes in PTEN -depleted cells as compared with wild-type cells ( Fig. 1a ). FANCD2 is a DNA damage marker that localizes as foci on mitotic chromosomes after replication fork stalling [16] , [17] . We therefore employed FANCD2 immunofluorescence to determine whether mitotic errors in PTEN -depleted cells result from the preceding S phase. Indeed, the majority of anaphase bridges as evaluated by a combination of DAPI and CENPA staining ( Fig. 1a ) are positive for FANCD2 ( Fig. 1b , Supplementary Fig. 1b ). More importantly, FANCD2-positive anaphase bridges appear at a remarkably increased frequency in cells containing PTEN-specific shRNA (shPTEN) (32.8% vs 12.9% as compared with control cells; Fig. 1b,c ). PTEN knockdown also significantly increases the number of FANCD2 bridges in each bridge-bearing anaphase cell ( Supplementary Fig. 1b ). These data illustrate that structural chromosomal aberrations arise through replication defects in cells depleted of PTEN . 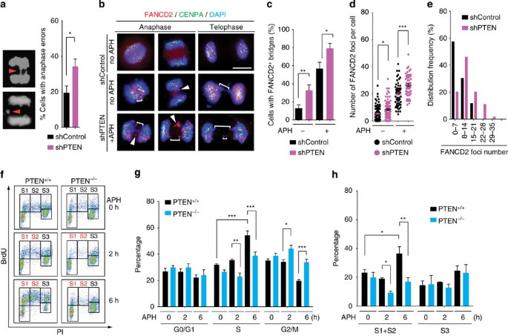Figure 1: PTEN depletion induces FANCD2-associated anaphase bridges and premature S phase exit. (a) Anaphase errors increase inPTEN-depleted cells. HeLa cells with and without PTEN shRNA (shPTEN and shControl,n=128 and 103, respectively) were examined by immunofluorescence for mitotic defects. Percentages of mitotic cells with anaphase bridges and micronuclei (arrowheads) are summarized in the histogram with represent 4,6-diamidino-2-phenylindole (DAPI) images shown on the left. Data are presented as means±s.e.m. and analysed by unpairedt-test. *P<0.05. (b) Specification of pre-mitotic errors originating from DNA replication barrier. Immunofluorescence of FANCD2 was employed for labelling damaged DNA in mitosis reflective of replication defects. CENPA and DAPI were used to indicate centromeres and chromosomes. Top panel; anaphase and telophase cells without prominent FANCD2 foci. Mid and bottom panels; cells in anaphase or telophase with pronounced FANCD2 foci. Brackets, paired foci; Arrowheads, single or accumulated foci; Scale bar, 5 μm. (c) Frequencies of FANCD2-associated ana-telophase bridges summarized from FANCD2 immunofluorescence in cells with or without shPTEN in the presence and absence of aphidicolin (APH) treatment (0.1 μM, 24 h). Data are presented as means±s.e.m. (n>50 for each column) and analysed by analysis of variance (ANOVA) with Turkey’s multiple comparisons test. *P<0.05; **P<0.01. (d) APH-treated HeLa cells with and without shPTEN were immunostained as inb. Mitotic cells were analysed for FANCD2 foci numbers and shown in a scatter plot. Data were processed by ANOVA and statistical significance was determined by Turkey’s multiple comparisons test. *P<0.05; ***P<0.001. (e) The distribution frequency of FANCD2 foci number in HeLa cells with and without shPTEN in the absence of APH treatment. (f)PTEN+/+andPTEN−/−DLD-1 cells were treated with 1 μM APH for 0, 2 or 6 h, before 5-bromo-2'-deoxyuridine (BrdU) labelling and propidium iodide (PI) staining for flow cytometry analysis of cell cycle distribution. S phase was divided into three sub-S phases (early-S1, mid-S2 and late-S3) as indicated. (g,h) Summaries of cell cycle distribution in different phases (G0/G1, S and G2/M,g) or sub-S phases (S1+S2 and S3,h), respectively. Figure 1: PTEN depletion induces FANCD2-associated anaphase bridges and premature S phase exit. ( a ) Anaphase errors increase in PTEN -depleted cells. HeLa cells with and without PTEN shRNA (shPTEN and shControl, n =128 and 103, respectively) were examined by immunofluorescence for mitotic defects. Percentages of mitotic cells with anaphase bridges and micronuclei (arrowheads) are summarized in the histogram with represent 4,6-diamidino-2-phenylindole (DAPI) images shown on the left. Data are presented as means±s.e.m. and analysed by unpaired t -test. * P <0.05. ( b ) Specification of pre-mitotic errors originating from DNA replication barrier. Immunofluorescence of FANCD2 was employed for labelling damaged DNA in mitosis reflective of replication defects. CENPA and DAPI were used to indicate centromeres and chromosomes. Top panel; anaphase and telophase cells without prominent FANCD2 foci. Mid and bottom panels; cells in anaphase or telophase with pronounced FANCD2 foci. Brackets, paired foci; Arrowheads, single or accumulated foci; Scale bar, 5 μm. ( c ) Frequencies of FANCD2-associated ana-telophase bridges summarized from FANCD2 immunofluorescence in cells with or without shPTEN in the presence and absence of aphidicolin (APH) treatment (0.1 μM, 24 h). Data are presented as means±s.e.m. ( n >50 for each column) and analysed by analysis of variance (ANOVA) with Turkey’s multiple comparisons test. * P <0.05; ** P <0.01. ( d ) APH-treated HeLa cells with and without shPTEN were immunostained as in b . Mitotic cells were analysed for FANCD2 foci numbers and shown in a scatter plot. Data were processed by ANOVA and statistical significance was determined by Turkey’s multiple comparisons test. * P <0.05; *** P <0.001. ( e ) The distribution frequency of FANCD2 foci number in HeLa cells with and without shPTEN in the absence of APH treatment. ( f ) PTEN +/+ and PTEN −/− DLD-1 cells were treated with 1 μM APH for 0, 2 or 6 h, before 5-bromo-2'-deoxyuridine (BrdU) labelling and propidium iodide (PI) staining for flow cytometry analysis of cell cycle distribution. S phase was divided into three sub-S phases (early-S1, mid-S2 and late-S3) as indicated. ( g , h ) Summaries of cell cycle distribution in different phases (G0/G1, S and G2/M, g ) or sub-S phases (S1+S2 and S3, h ), respectively. Full size image Aphidicolin (APH) is a DNA polymerase inhibitor that causes the replication fork to stall and potentially collapse; FANCD2 specifically targets replication stress-induced chromatid gaps and breaks [16] . We therefore treated cells with APH and compared the frequency of FANCD2-positive anaphase bridges. APH treatment dramatically increases the frequency of cells with FANCD2-labelled anaphase bridges even in wild-type cells (56.9% vs 12.9%; Fig. 1c ), further confirming that these mitotic errors originate from aberrant replication intermediates. As FANCD2 foci are usually found on chromatin arms [17] , it is believed that the FANC pathway repairs non-centromeric abnormal structures induced by replication stress [16] , [18] . However, we noticed that sister foci of FANCD2 often overlap or localize in close proximity with CENPA foci ( Supplementary Fig. 1c ), suggesting that FANCD2-labelled DNA damage is not limited to non-centromeric regions. Although the source and number of FANCD2 foci vary, the foci found in mitotic cells reflect replication-originating DNA damage [18] . PTEN -depleted mitotic cells have an increased number of FANCD2 foci than wild-type cells even in the absence of APH treatment ( Fig. 1d ). APH significantly enhances the difference between PTEN knockdown cells and control cells ( Fig. 1d , Supplementary Fig. 1d ), suggesting a reduced capability of PTEN -depleted cells to overcome DNA damage, likely due to impairment of the replication machinery. The distribution frequencies of FANCD2 foci number further illustrate the increased obstacle of DNA replication in cells lacking PTEN ( Fig. 1e and Supplementary Fig. 1d ). Taken together, these data suggest that depletion of PTEN induces spontaneous DNA replication errors that result in chromosome entanglement and subsequent segregation defects, which can be further aggravated by exogenous replication perturbation. Loss of PTEN confers replication stress tolerance Impaired DNA replication normally activates the replication checkpoint causing an S phase delay. We therefore anticipated that endogenous replication defects would arrest PTEN -deficient cells in S phase. However, BrdU (5-bromo-2'-deoxyuridine) labeling and flow cytometry analysis showed a slight S phase reduction in PTEN null cells, which becomes increasingly significant when cells are challenged with APH over a time course ( Fig. 1f,g ). These results suggest that endogenous replication defects in PTEN -deficient cells ( Fig. 1a–e ) are insufficient to activate the replication checkpoint and that the checkpoint may become less responsive even in response to exogenous replication perturbation. Alternatively, these cells have acquired an adaptation to chronic endogenous replication stress and even to acute exogenous replication inhibition. In wild-type cells, 2-h treatment with a low dose of APH is insufficient to induce S phase arrest, whereas a dramatic checkpoint response, as manifested by S phase arrest, occurs at 6 h following APH treatment ( Fig. 1f,g ). At both time points, PTEN -null cells exhibit a significant reduction of the S phase population as compared with wild-type control cells ( Fig. 1g ). Corresponding to the S phase reduction, remarkably higher percentages of PTEN -null cells accumulate in G2/M phases as compared with wild-type cells at each time point. These data suggest that PTEN -null cells acquire a mechanism to escape the APH-mediated replication barrier in a checkpoint-independent manner. These results support the idea of a replication stress tolerance mechanism that may be adopted by PTEN -depleted cells to ignore or bypass replication-derived DNA lesions. As a consequence, these cells exit S phase with incomplete or faulty DNA replication and proceed prematurely into M phase with replication-derived mitotic errors, such as the FANCD2 anaphase bridges we observed in Fig. 1a–e . To further determine which specific stage of S phase is affected by PTEN depletion, we divided the S phase population into three sub-populations: early, mid and late S phases ( Fig. 1f ). The most prominent difference in the S phase distribution occurs in early or mid S phases (S1 or S1+S2, Fig. 1h ), suggesting that the replication in early S phase is preferentially protected by PTEN. These observations have been confirmed in PTEN knockdown HeLa cells using different replication inhibitors including APH and hydroxyurea (HU, Supplementary Fig. 1e–g ). PTEN depletion elevates endogenous replication stress To better understand the impact of PTEN loss on DNA replication, we used a DNA fibre technique to visualize replication origin firing, fork progression and recovery from stalled forks at the single molecule level. To monitor natural dynamics of replication forks, we first pulse labelled PTEN +/+ and PTEN −/− DLD-1 cells in unperturbed S phase with nucleotide analogue CldU (5-Chloro-2’-deoxyuridine) and traced nascent replication tracts on single-strand DNA (ssDNA, Fig. 2a ). The use of an asynchronous cell population avoids any artifacts introduced by synchronization procedures. We observed overall longer CldU tracts in wild-type cells as compared with PTEN -null cells (12.32±6.24 vs 8.90±4.26 μm, Fig. 2b ). After 30 min of labelling, wild-type cells had CldU tract lengths mostly over 13.5 μm, while PTEN -null cells had much shorter tracts, mostly under 8.5 μm ( Fig. 2c ). These results indicate a slower fork progression rate in PTEN -null cells, which may also be interpreted as a higher frequency of fork stalling or a delay in the clearance of stalled forks. Any condition that results in replication fork slowing or stalling is counteracted by local increases in origin density [19] . Indeed, the average inter-origin distance is significantly reduced upon PTEN deletion ( Fig. 2d ), suggesting that a higher frequency of stalled forks induces compensatory activation of dormant origins. 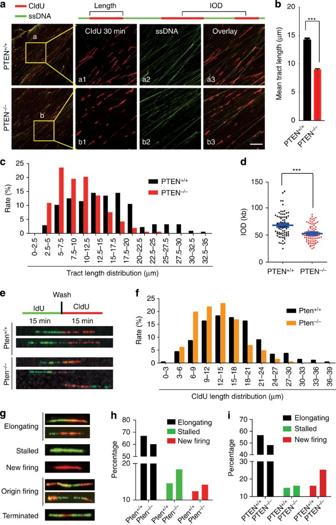Figure 2: Replication fork progression is impaired in the absence of PTEN. (a)PTEN+/+andPTEN−/−DLD-1 cells were pulse-labelled with CldU and subjected to single DNA fibre analysis. CldU tracts were visualized in red and ssDNA in green. Above the images is a schematic of the assay and data shown are from a single representative experiment out of three repeats. Scale bar, 25 μm. (b) Summary of mean CldU tract length inPTEN-proficient (n=302) and -deficient (n=301) cells. Data are presented as means±s.e.m. and analysed by unpairedt-test. ***P<0.001. (c) CldU fibre tract length distributions inPTEN+/+andPTEN−/−cells. 1 μm=2 kb. (d) Distributions of the inter-origin distances (IOD) inPTEN+/+andPTEN−/−cells. IOD was determined by measuring the distance between two identified replication initiation origins, as indicated by the sketch ina. Bars and error bars represent means±s.e.m. (n>75 in each cell group); ***P<0.001. (e,f)Pten+/+andPten−/−MEFs were sequentially pulse-labelled with 50 μM IdU and 50 μM CldU, each for 15 min. Green tracts, IdU; Red tracts, CldU. A sketch delineating experimental design and representative images of dual-labelled fibres are shown ine. Second-labelled CldU tract length distributions inPten+/+(n=302) andPten−/−(n=300) cells are shown inf. (g) Examples of fibre tract types representing different classes of replication structures. (h,i) Replication profiles ofPTEN-proficient and -deficient MEFs (h) and DLD-1 cells (i) are presented by scoring relative frequencies of elongating fibres versus stalled or new-fired fibres. Minimums of 300 fibres were scored in each cell line. Figure 2: Replication fork progression is impaired in the absence of PTEN. ( a ) PTEN +/+ and PTEN −/− DLD-1 cells were pulse-labelled with CldU and subjected to single DNA fibre analysis. CldU tracts were visualized in red and ssDNA in green. Above the images is a schematic of the assay and data shown are from a single representative experiment out of three repeats. Scale bar, 25 μm. ( b ) Summary of mean CldU tract length in PTEN -proficient ( n =302) and -deficient ( n =301) cells. Data are presented as means±s.e.m. and analysed by unpaired t -test. *** P <0.001. ( c ) CldU fibre tract length distributions in PTEN +/+ and PTEN −/− cells. 1 μm=2 kb. ( d ) Distributions of the inter-origin distances (IOD) in PTEN +/+ and PTEN −/− cells. IOD was determined by measuring the distance between two identified replication initiation origins, as indicated by the sketch in a . Bars and error bars represent means±s.e.m. ( n >75 in each cell group); *** P <0.001. ( e , f ) Pten +/+ and Pten −/− MEFs were sequentially pulse-labelled with 50 μM IdU and 50 μM CldU, each for 15 min. Green tracts, IdU; Red tracts, CldU. A sketch delineating experimental design and representative images of dual-labelled fibres are shown in e . Second-labelled CldU tract length distributions in Pten +/+ ( n =302) and Pten −/− ( n =300) cells are shown in f . ( g ) Examples of fibre tract types representing different classes of replication structures. ( h , i ) Replication profiles of PTEN -proficient and -deficient MEFs ( h ) and DLD-1 cells ( i ) are presented by scoring relative frequencies of elongating fibres versus stalled or new-fired fibres. Minimums of 300 fibres were scored in each cell line. Full size image The relatively slower replication in PTEN -null cells could also reflect an extended pausing at natural pause sites. To exclude the interference by the possible fusion of converging replication forks, we employed a consecutive dual labelling approach to label DNA fibres with two different nucleotide analogues that can be distinguished with specific antibodies. Measurement of second-labelled DNA fibres revealed a significant decrease in CldU tract lengths in Pten −/− mouse embryo fibroblasts (MEFs) as compared with Pten +/+ cells ( Fig. 2e ). The mean tract length of CldU and the frequency distribution in MEF, DLD-1 and HeLa ( Fig. 2f and Supplementary Fig. 2a–e ) mirror each other and collectively corroborate that PTEN protects continuous DNA synthesis. These data suggest that in the absence of PTEN, replication forks undergo an intrinsically unsteady progression, and experience more frequent pauses than programmed at natural pause sites. Together, these results demonstrate that PTEN functions during DNA replication to facilitate fork progression and that loss of PTEN leads to fork slowing or stalling even in the absence of exogenous sources of replication stress. The dual labelling protocol also allows classification of five major patterns of the replication profile, as individually depicted in Fig. 2g . Based on this classification, we analysed the replication profile in multiple PTEN -deficient cell systems and observed consistent alterations. As shown in Fig. 2h,i , a reduced proportion of PTEN -null cells display normal replication progression (elongating type), whereas stalled and new firing replication forks occur more frequently in cells lacking PTEN. These data further confirm that, on a global scale, PTEN deficiency impairs replication fork progression and alters replication dynamics. Slowing or stalling replication forks in PTEN -deficient cells represent a spontaneous source of endogenous replication stress. PTEN is required for reactivation of stalled forks Having found that spontaneous replication-associated DNA damage in PTEN knockdown cells is further aggravated by APH treatment, we proceeded to examine how endogenous replication stress incurred by PTEN loss affects cellular response to acute exogenous replication perturbation. We used a modified double labelling method by pre-labelling cells with CldU before HU or APH treatment and assessed fork recovery through second labelling of IdU (5-Iodo-2’-deoxyuridine; Fig. 3a ). In wild-type cells, the majority of forks are able to resume DNA synthesis, manifested by red–green tracts ( Fig. 3b ). In contrast, PTEN -null cells exhibit a dramatically increased frequency of stalled forks (red tracts only), as summarized in Fig. 3c . Interestingly, we noticed that a large portion of red–green tracts in PTEN −/− cells have gaps between the two-colour labelling (55%), whereas this occurs rarely (3.8%) in wild-type cells. Moreover, the gaps in red–green tracts are significantly larger in PTEN −/− cells (2.1 μm) than in PTEN +/+ cells (0.8 μm, Fig. 3d ). These gaps are likely formed by stalled forks and nearby newly fired origins initiated after release from HU. Similar to HU, APH treatment causes a higher frequency of stalled forks in PTEN −/− DLD-1 cells ( Fig. 3e ). Pten −/− MEFs also exhibit a higher sensitivity to HU- or APH-induced replication fork stalling as compared with wild-type cells ( Fig. 3f ). These results jointly demonstrate that PTEN plays a general and essential role in stalled replication fork recovery following exogenous replication perturbation. 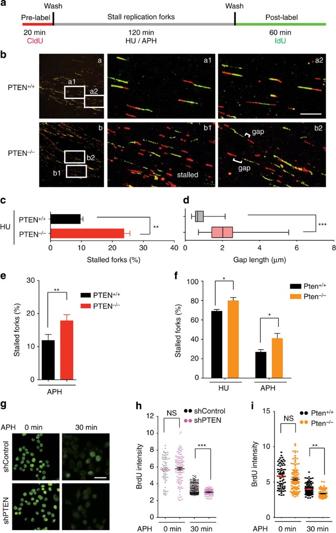Figure 3: PTEN is required for restart of DNA replication at stalled forks. (a) A schematic protocol of dual labelling DNA fibre assay for evaluation of replication restart following HU- or APH-induced fork stalling. (b)PTEN+/+andPTEN−/−DLD-1 cells were pre-labelled with CldU and then treated with 2 mM HU for 2 h, before post-labelling with IdU for monitoring replication recovery. Selected areas are magnified for visual enhancement of stalled CldU tracts and gaps between CldU and IdU tracts in PTEN-null cells. Scale bar, 10 μm. (c,d) Summary of stalled fork frequencies (n>300) and gap lengths (n>200) between stalled sites and their corresponding re-initiation sites. Data are presented as means±s.e.m. and analysed by unpairedt-test. **P<0.01; ***P<0.001. (e) Summary of DNA fibre restart assay inPTEN+/+(n=284) andPTEN−/−(n=336) cells following APH (3 μM) treatment. Data were scored and analysed as ind. **P<0.01. (f)Pten+/+andPten−/−MEFs were pulse labelled with CldU and subsequently treated with HU (2 mM) or APH (3 μM) for 2 h, followed by IdU pulse labelling to monitor replication recovery. A minimum of 200 fibre units was scored for each criterion. Data are presented as means±s.e.m. and analysed by unpairedt-test. *P<0.05. (g) BrdU incorporation analysis in response to APH treatment. HeLa cells with and without shRNA-mediatedPTENknockdown were subjected to 3 μM APH treatment for different time periods as indicated, before BrdU pulse labelling for 15 min. Cells were then fixed for immunofluorescence of BrdU. Scale bar, 25 μm. (h) Immunofluorescence images fromgwere analysed for BrdU intensity and summarized as mean intensity per cell (n>150). Data are presented as means±s.e.m. in relative arbitrary unit and analysed by unpairedt-test. NS, not significant; ***P<0.001. (i)Pten+/+andPten−/−MEFs were treated with 3 μM APH for 30 min followed by BrdU pulse labelling. Immunofluorescence intensities of BrdU were scored before and after APH treatment. Data were analysed by analysis of variance and statistical significance was determined by Turkey’s multiple comparison tests. **P<0.01. Figure 3: PTEN is required for restart of DNA replication at stalled forks. ( a ) A schematic protocol of dual labelling DNA fibre assay for evaluation of replication restart following HU- or APH-induced fork stalling. ( b ) PTEN +/+ and PTEN −/− DLD-1 cells were pre-labelled with CldU and then treated with 2 mM HU for 2 h, before post-labelling with IdU for monitoring replication recovery. Selected areas are magnified for visual enhancement of stalled CldU tracts and gaps between CldU and IdU tracts in PTEN-null cells. Scale bar, 10 μm. ( c , d ) Summary of stalled fork frequencies ( n >300) and gap lengths ( n >200) between stalled sites and their corresponding re-initiation sites. Data are presented as means±s.e.m. and analysed by unpaired t -test. ** P <0.01; *** P <0.001. ( e ) Summary of DNA fibre restart assay in PTEN +/+ ( n =284) and PTEN −/− ( n =336) cells following APH (3 μM) treatment. Data were scored and analysed as in d . ** P <0.01. ( f ) Pten +/+ and Pten −/− MEFs were pulse labelled with CldU and subsequently treated with HU (2 mM) or APH (3 μM) for 2 h, followed by IdU pulse labelling to monitor replication recovery. A minimum of 200 fibre units was scored for each criterion. Data are presented as means±s.e.m. and analysed by unpaired t -test. * P <0.05. ( g ) BrdU incorporation analysis in response to APH treatment. HeLa cells with and without shRNA-mediated PTEN knockdown were subjected to 3 μM APH treatment for different time periods as indicated, before BrdU pulse labelling for 15 min. Cells were then fixed for immunofluorescence of BrdU. Scale bar, 25 μm. ( h ) Immunofluorescence images from g were analysed for BrdU intensity and summarized as mean intensity per cell ( n >150). Data are presented as means±s.e.m. in relative arbitrary unit and analysed by unpaired t -test. NS, not significant; *** P <0.001. ( i ) Pten +/+ and Pten −/− MEFs were treated with 3 μM APH for 30 min followed by BrdU pulse labelling. Immunofluorescence intensities of BrdU were scored before and after APH treatment. Data were analysed by analysis of variance and statistical significance was determined by Turkey’s multiple comparison tests. ** P <0.01. Full size image Difficulty resuming stalled forks may directly result from chromosome fragility and vulnerability to stress-induced DNA lesions. To further consolidate the increased sensitivity of PTEN -depleted cells to APH-mediated inactivation of replication forks, we examined BrdU incorporation in pulse-labelled cells with and without shPTEN following APH treatment. While the amount of basal BrdU incorporation is similar in cells with and without PTEN knockdown, APH treatment reduces BrdU incorporation in PTEN knockdown cells to a significantly greater extent ( Fig. 3g,h ), indicating that stalled replication fork recovery is less effective in the absence of PTEN. We also confirmed these observations in Pten -null MEFs ( Fig. 3i ). This is in agreement with the S phase reduction as observed in cells with PTEN depletion ( Fig. 1f–h and Supplementary Fig. 1e–g ). PTEN maintains key replication factors on chromatin The whole process of DNA replication, including initiation, progression and recovery, takes place on chromatin and requires spatial coordination of a large number of protein regulators [20] . Our recent work pointed to the interplay of PTEN with histones in the maintenance of chromatin condensation [5] . It is thus plausible that PTEN loss-induced chromatin decondensation may affect local replication activity. We therefore performed a fractionation procedure to examine important replication factors in different cellular fractions. We found that chromatin-associated Rad51, PCNA and Chk1 are significantly reduced in PTEN knockout cells ( Fig. 4a ). Histone deacetylase inhibitor trichostatin A (TSA) can mimic PTEN depletion to cause chromatin decondensation and dissociation of histone H1 from chromatin [5] . In accordance, we observed chromatin dissociation of Rad51, PCNA and Chk1 in TSA-treated cells ( Fig. 4b ), suggesting a role of condensed chromatin in facilitating chromatin recruitment of important replication factors. These data also imply that in the absence of replication stress, PTEN function in chromatin compaction is necessary for the maintenance of replication regulators on chromatin. 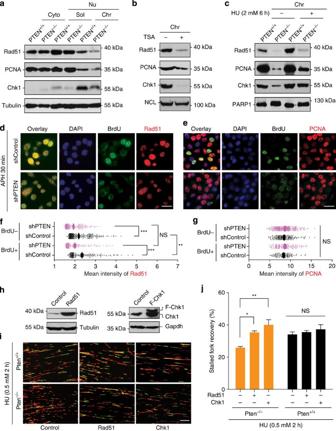Figure 4: PTEN maintains replication proteins on chromatin for stalled fork recovery. (a) Cellular fractionation was performed inPTEN-proficient or -deficient DLD-1 cells to separate cytoplasm soluble fraction, nuclear-soluble fraction and chromatin fraction, as described in Methods. Protein lysates from different fractions were immunoblotted with Rad51, PCNA and Chk1 antibodies. Tubulin was used as a loading control. (b)PTEN+/+DLD-1 cells were subjected to trichostatin A (TSA) treatment (10 μM, 12 h) followed by chromatin isolation for western analysis of Rad51, PCNA and Chk1, respectively. (c) Levels of Rad51, PCNA and Chk1 were evaluated with immunoblotting using chromatin fractions fromPTEN+/+andPTEN−/−DLD-1 cells in the presence and absence of HU treatment. (d,e) APH-treated PTEN knockdown and control cells were pulse labelled with BrdU followed by Rad51 and PCNA immunofluorescence. Scale bar, 25 μm. (f,g) Immunofluorescent intensity of Rad51 (d) and PCNA (e) was quantified and summarized in BrdU-positive and -negative categories. One-way analysis of variance (ANOVA) was used for statistical analysis and Bonferroni’s multiple comparison tests were used for evaluation of statistical significance. **P<0.01; ***P<0.001. NS, not significant. (h) Western blots to show overexpression of Rad51 or FLAG-tagged Chk1 inPten−/−MEFs. (i)Pten+/+andPten−/−MEFs were pre-labelled with CldU and then treated with 0.5 mM HU for 2 h, before post-labelling with IdU for monitoring replication recovery. Shown is representative DNA fibre images of indicated samples. Scale bar, 25 μm. (j) Summary of DNA stalled fork restart inPten+/+andPten−/−cells with and without ectopic Rad51 or Chk1 following HU treatment (n>1,000 in each sample). Data were analysed with one-way ANOVA followed by Turkey’s multiple comparison tests. *P<0.05; **P<0.01. Figure 4: PTEN maintains replication proteins on chromatin for stalled fork recovery. ( a ) Cellular fractionation was performed in PTEN -proficient or -deficient DLD-1 cells to separate cytoplasm soluble fraction, nuclear-soluble fraction and chromatin fraction, as described in Methods. Protein lysates from different fractions were immunoblotted with Rad51, PCNA and Chk1 antibodies. Tubulin was used as a loading control. ( b ) PTEN +/+ DLD-1 cells were subjected to trichostatin A (TSA) treatment (10 μM, 12 h) followed by chromatin isolation for western analysis of Rad51, PCNA and Chk1, respectively. ( c ) Levels of Rad51, PCNA and Chk1 were evaluated with immunoblotting using chromatin fractions from PTEN +/+ and PTEN −/− DLD-1 cells in the presence and absence of HU treatment. ( d , e ) APH-treated PTEN knockdown and control cells were pulse labelled with BrdU followed by Rad51 and PCNA immunofluorescence. Scale bar, 25 μm. ( f , g ) Immunofluorescent intensity of Rad51 ( d ) and PCNA ( e ) was quantified and summarized in BrdU-positive and -negative categories. One-way analysis of variance (ANOVA) was used for statistical analysis and Bonferroni’s multiple comparison tests were used for evaluation of statistical significance. ** P <0.01; *** P <0.001. NS, not significant. ( h ) Western blots to show overexpression of Rad51 or FLAG-tagged Chk1 in Pten −/− MEFs. ( i ) Pten +/+ and Pten −/− MEFs were pre-labelled with CldU and then treated with 0.5 mM HU for 2 h, before post-labelling with IdU for monitoring replication recovery. Shown is representative DNA fibre images of indicated samples. Scale bar, 25 μm. ( j ) Summary of DNA stalled fork restart in Pten +/+ and Pten −/− cells with and without ectopic Rad51 or Chk1 following HU treatment ( n >1,000 in each sample). Data were analysed with one-way ANOVA followed by Turkey’s multiple comparison tests. * P <0.05; ** P <0.01. Full size image We next investigated how exogenous replication stress might affect chromatin anchorage of replication regulators in the presence and absence of PTEN. HU treatment induces chromatin loading of Rad51 in wild-type cells, which is dramatically dampened in the absence of PTEN ( Fig. 4c ). Due to a higher basal chromatin level of PCNA and Chk1 in PTEN +/+ cells, HU only slightly increases further chromatin association of Chk1, to an even minor extent, of PCNA. In contrast, PTEN −/− cells, with a lower basal level of PCNA and Chk1 on chromatin, exhibit a more significant chromatin recruitment of both proteins in response to HU treatment ( Fig. 4c ). To determine how different patterns of chromatin loading may affect the involvement of these key regulators in the PTEN replication pathway, we compared the correlation of Rad51 or PCNA with BrdU incorporation in pulse-labelled cells following APH treatment. Rad51 displays a homogeneous staining pattern without discrete foci formation ( Fig. 4d ), consistent with the previous report that Rad51 mediates replication fork recovery without necessarily forming foci at stalled replication forks [21] . We found that replicating cells (BrdU positive) exhibit a higher intensity of Rad51 ( Fig. 4d ). However, there is no correlation between PCNA intensity and BrdU incorporation ( Fig. 4e ). More interestingly, Rad51 no longer correlates with BrdU in PTEN knockdown cells ( Fig. 4f ), suggesting that loss of PTEN decouples Rad51 function from replication recovery. Nevertheless, the corresponding relationship between PTEN status and Rad51 signal intensity, for example, lower intensities of Rad51 in cells deficient of PTEN , appears to be constant even in the BrdU-negative category ( Fig. 4f ). These data highlight a functional link between PTEN and Rad51 in replication recovery. In contrast, PTEN status does not affect PCNA signal intensities in APH-treated cells ( Fig. 4g ). As a DNA sliding clamp in the basal replication machinery [22] , PCNA may play a role in PTEN-dependent maintenance of replication fork stability without involving stress-responsive replication recovery. While PCNA functions primarily to maintain the basal replication machinery, Rad51 and Chk1 are better known for stalled fork stabilization and repair in the presence of replication stress [23] . To evaluate the capability of Rad51 and Chk1 in promoting the restart of stalled forks in PTEN -deficient cells, we performed CldU–IdU dual labelling and examined DNA fibres following HU treatment in cells overexpressing Rad51 or Chk1, respectively. As shown in Fig. 4h–j , ectopic Rad51 and Chk1 can both significantly enhance the recovery of HU-stalled replication forks in Pten −/− cells. When we repeated these experiments in Pten +/+ cells, overexpression of neither Rad51 nor Chk1 showed significant improvement of fork recovery. Similarly in APH-treated cells, Rad51 significantly induced fork recovery in Pten −/− cells but not in Pten +/+ cells ( Supplementary Fig. 3 ). These results suggest that PTEN may act epistatically with either Rad51 or Chk1 in facilitating stalled fork restart in response to exogenous replication stress. PTEN acts on DNA replication forks to recruit Rad51 Recent studies have expanded the concept of nuclear PTEN by revealing its physical association with diverse nuclear apparatus including centromeres [2] and centrosomes [11] . We have also demonstrated the interplay of PTEN with histones on chromatin [5] . To determine whether PTEN itself can respond to replication stress, we treated both PTEN +/+ and PTEN −/− cells with HU and examined PTEN protein levels in the chromatin fraction. We found that HU induces PTEN loading on chromatin in a time-dependent manner ( Fig. 5a ). In addition, PTEN can physically interact with both Rad51 and Chk1 following HU treatment ( Fig. 5b ). To scrutinize how these proteins coordinate in response to replication stress, we employed a high-resolution iPOND ( I solation of P rotein O n N ascent D NA) technique [24] to examine the spatiotemporal relationship of PTEN with Rad51 and Chk1 specifically on DNA replication forks. Our data first uncovered the physical localization of PTEN on stalled replication forks and the enhancement of its fork recruitment following HU treatment ( Fig. 5c ). As our input samples are nuclear fractions, the higher level of PTEN input in the HU-treated PTEN +/+ cells reflects an increased nuclear import. In addition to PTEN loading on HU-stalled replication forks, we also observed a similar fork-recruitment pattern of Rad51 following HU-induced replication stress. The Chk1 level on stalled replication forks, however, does not appear to be significantly altered by either the PTEN status or HU treatment ( Fig. 5c ). These data suggest that a substantial amount of Chk1 is constantly associated with replication forks even in the absence of PTEN or exogenous replication stress. Although exogenous replication stress can induce PTEN interaction with Rad51 and Chk1 ( Fig. 5b ), loss of PTEN leads to replication fork dissociation of Rad51, but not Chk1, as depicted in Fig. 5d . Therefore, the epistatic relationship may only apply between PTEN and Rad51 during stalled fork recovery. 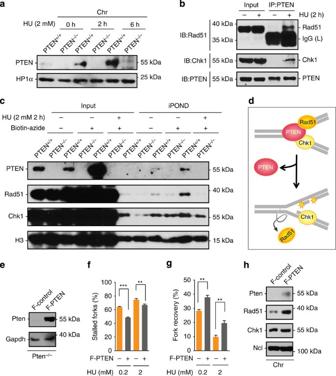Figure 5: PTEN is physically associated with DNA replication forks and PTEN recruits Rad51 on chromatin for stalled fork recovery. (a) Chromatin was isolated fromPTEN+/+andPTEN−/−DLD-1 cells in the presence and absence of 2 mM HU for indicated time periods, before PTEN immunoblotting. (b) Cell lysates were prepared fromPTEN+/+DLD-1 cells following sonication-induced chromatin lysis. Cells with and without HU treatment (2 mM, 2 h) were subjected to PTEN immunoprecipitation followed by immunoblotting of Rad51 and Chk1. (c)PTEN+/+andPTEN−/−HCT116 cells were labelled with EdU and treated with 2 mM HU. Nascent DNA was conjugated with biotin for iPOND analysis as described in Methods. DNA replication fork-associated PTEN, Rad51 and Chk1 were detected by western blotting. Histone H3 was used a loading control. (d) A schematic model to show formation of the PTEN-Rad51-Chk1 complex on DNA replication forks in normal conditions and Rad51 dissociation (Chk1 may retain) following PTEN depletion. (e) PTEN overexpression inPten−/−MEFs. (f,g)Pten−/−MEFs containing ectopic PTEN were treated with different doses of HU, before sequential IdU-CldU pulse labelling. The frequency of stalled forks and fork restart (stalled and elongating type as depicted inFig. 2g) was scored. Data are presented as means±s.e.m. and analysed with unpairedt-test. **P<0.01; ***P<0.001. (h)Pten−/−MEFs with and without ectopic PTEN were subjected to isolation of chromatin fraction, followed by western analysis of Pten, Rad51 and Chk1. Ncl was used to indicate equal loading of chromatin fractions. Figure 5: PTEN is physically associated with DNA replication forks and PTEN recruits Rad51 on chromatin for stalled fork recovery. ( a ) Chromatin was isolated from PTEN +/+ and PTEN −/− DLD-1 cells in the presence and absence of 2 mM HU for indicated time periods, before PTEN immunoblotting. ( b ) Cell lysates were prepared from PTEN +/+ DLD-1 cells following sonication-induced chromatin lysis. Cells with and without HU treatment (2 mM, 2 h) were subjected to PTEN immunoprecipitation followed by immunoblotting of Rad51 and Chk1. ( c ) PTEN +/+ and PTEN −/− HCT116 cells were labelled with EdU and treated with 2 mM HU. Nascent DNA was conjugated with biotin for iPOND analysis as described in Methods. DNA replication fork-associated PTEN, Rad51 and Chk1 were detected by western blotting. Histone H3 was used a loading control. ( d ) A schematic model to show formation of the PTEN-Rad51-Chk1 complex on DNA replication forks in normal conditions and Rad51 dissociation (Chk1 may retain) following PTEN depletion. ( e ) PTEN overexpression in Pten −/− MEFs. ( f , g ) Pten −/− MEFs containing ectopic PTEN were treated with different doses of HU, before sequential IdU-CldU pulse labelling. The frequency of stalled forks and fork restart (stalled and elongating type as depicted in Fig. 2g ) was scored. Data are presented as means±s.e.m. and analysed with unpaired t- test. ** P <0.01; *** P <0.001. ( h ) Pten −/− MEFs with and without ectopic PTEN were subjected to isolation of chromatin fraction, followed by western analysis of Pten, Rad51 and Chk1. Ncl was used to indicate equal loading of chromatin fractions. Full size image To interrogate the functional interplay between PTEN and Rad51 in facilitating replication fork restart, we transfected Pten −/− MEFs with PTEN or Rad51 and compared their replication profiles in response to HU or APH treatment. As shown in Supplementary Fig. 4 , both PTEN and Rad51 similarly reduce the frequency of stalled forks, mainly through the induction of replication fork restart. The impairment of fork recovery under replication stress in PTEN -deficient cells can be rescued by restoration of PTEN expression ( Fig. 5e–g ). Interestingly, PTEN overexpression results in an increased chromatin loading of Rad51 but not of Chk1 ( Fig. 5h ), further validating the PTEN-Rad51 signalling axis in promoting DNA replication fork stability. Rad51 may also serve as a limiting factor in resumption of stalled forks. Indeed, we found a prominent reduction of chromatin-bound Rad51 in PTEN -null cells following APH treatment ( Supplementary Fig. 5a ), indicating diminished availability of Rad51 for replication stress response. Pten -null cells exhibit a reduced level of Rad51 on chromatin for 12 h following APH treatment ( Supplementary Fig. 5b , 0–12 h). A prolonged treatment with APH (24 h) is able to induce Rad51 in both Pten +/+ and Pten −/− cells to a similar level, which may be responsible for HR-mediated DNA repair. These data suggest that chromatin-bound Rad51 may represent a local repository of Rad51, insufficiency of which compromises the initiation and progression of replication forks under replication stress. DNA replication is the central event during inheritance of the genetic information and PTEN is a powerful tumour suppressor with known functions in guarding the genome. In this study, we elucidate the importance of PTEN in protecting the replication process. Our data reveal two aspects of PTEN function in DNA replication under unperturbed or perturbed conditions, both associated with the term ‘replication stress’ despite distinct phenotypes. First, in the absence of exogenous challenge, loss of PTEN results in spontaneous impairment of replication fork progression and alteration of replication dynamics. This phenotype reflects an endogenous replication stress status. Second, in the presence of exogenous challenge via replication inhibitors, PTEN loss compromises the efficiency of stalled replication folk resumption and the integrity of the replication checkpoint or checkpoint response. This may represent worsening of replication stress or deterioration of the endogenously impaired replication machinery. Acute exogenous replication stress by APH or HU usually affects one cell cycle and causes discrete pause sites locally. In contrast, depletion of PTEN results in a chronic and continuous stress condition through every cell cycle that globally affects the inherent replication machinery and dynamics. Progressive accumulation of replication errors, in line with acquired damage tolerance, may thereby form a cascade of replication stress leading to genomic instability in cells lacking PTEN. Replication stress reflects chromosome fragility and, therefore, common fragile site instability is a sensitive readout for replication stress [25] . Phosphorylation of H2AX on S139 (γ-H2AX) is a well-characterized early marker of DNA damage and is frequently used as a replication stress maker [26] . Retrospectively, many of our previous observations provide additional evidence for endogenous replication stress in PTEN -deficient cells. For example, our recent report demonstrated that deletion of Pten or its C-terminal region leads to increased number of γ-H2AX foci. In addition, common fragile site rearrangement was also observed in cells lacking the Pten C-terminal region [15] . Common fragile sites stability relies on efficient replication fork progression and recovery [27] ; it is thus conceivable that Pten mutant cells with impaired replication control mechanisms fail to maintain faithful replication of fragile sequences. Multiple forms of genomic instability including replication defects may contribute to the development of multiple tumours in mice lacking Pten . Loss of PTEN induces endogenous replication stress under normal conditions and causes replication stress tolerance in the presence of exogenous acute replication stress. Rad51 plays multiple roles in the cellular response to replication stress; Rad51 facilitates replication fork restart when forks are viable, repair of fork-associated DNA damage after forks have collapsed and firing of new origins for global replication rescue [21] . In addition to DNA replication, Rad51 also functions in damage repair primarily through homologous recombination (HR) and the formation of Rad51 nucleofilaments or foci indicates activation of the HR pathway [28] . Recent studies reveal a HR-independent replication restart pathway of Rad51 during replication stress [21] , which may contribute to PTEN function in replication. Our immunofluorescence data show that Rad51 exhibits a ubiquitous distribution without forming discrete foci, suggesting that loss of PTEN is associated with a reduction of chromatin-bound Rad51, likely in an HR-inactivated microenvironment. We previously reported that PTEN regulates Rad51 expression for HR-mediated double strand break repair [2] . Follow-up studies generated mixed results [3] , [29] , [30] , [31] , suggesting that the overall expression level of Rad51 is a combined consequence of multiple regulatory mechanisms. Data in this study advance previous observations by pinpointing the regulatory relationship between PTEN and Rad51 specifically at DNA replication forks within a chromatin microenvironment. PTEN-dependent chromatin loading of Rad51 and replication fork association offers a novel and reliable signalling marker for PTEN nuclear function. This study demonstrates that PTEN induces the recruitment of Rad51 on chromatin and accommodates its local accessibility to stalled replication forks for restart. These data highlight the PTEN–Rad51 axis in signalling cellular response to replication stress to ensure high efficiency and fidelity of DNA replication. Together, our findings suggest that PTEN controls critical cellular processes for faithful genome transmission through multiple mechanisms. Cell culture and reagents Pten +/+ and Pten −/− MEFs (provided by P.P. Pandolfi, Harvard Medical School), PTEN +/+ and PTEN −/− HCT116 cells (a kind gift from T. Waldman, Georgetown University), PTEN +/+ and PTEN −/− DLD-1 cells (from Sigma-Aldrich) and HeLa cells (from ATCC) were cultured in MEM supplemented with 10% fetal bovine serum. The pSUPER RNAi system (Oligoengine Inc.) was used to construct PTEN-specific shRNA expression plasmids and scrambled control shRNA. PTEN, Rad51 and Chk1 expression plasmids were constructed in a pCMV expression vector. BrdU, IdU, CldU, APH and HU were from Sigma-Aldrich. The following antibodies were used: PTEN (A2B1), Rad51 (H92), PCNA (FL-261), Chk1 (G4), PARP1/2 (H250), β -actin antibodies from Santa Cruz; BrdU from BD Pharmingen; CENPA and anti-ssDNA from EMD Millipore; Rat anti-BrdU BU1/75 and FANCD2 from Novus; FLAG (M2–3165) from Sigma-Aldrich. Immunofluorescence and microscopy Cells grown on glass slides were fixed and permeabilized for immunofluorescence. After blocking, cells were stained with single or combined primary antibodies for 2 h at room temperature then with Alexa Fluor-conjugated secondary antibody (Invitrogen) for 30 min. Images were acquired using a Nikon Eclipse TiE microscope. Images were acquired as z -stacks with 0.2–0.4 μm spacing to generate maximum-intensity projection of the entire cell. Imaging data were analysed using the NIS-Elements AR software. BrdU incorporation and cell cycle analysis Cells were pretreated with APH or HU and subsequently labelled with 50 μM BrdU for 20 min. Samples were immunostained with mouse anti-BrdU (BD Pharmingen) according to the manufacturer’s instructions and subjected to analysis using a FACScan (BD) cytometer. Data were analysed using FlowJo software (Tree Star). DNA fibre analysis Analysis of replicating DNA were performed according to the methods described previously [32] . In brief, cells were pulse-labelled with 50 μM CldU for 15 min, followed by second labelling with 50 μM IdU for 15 min before analysis. Cells were harvested and DNA fibres were stretched onto glass slides in a DNA lysis buffer (200 mM Tris-HCl at pH 7.4, 0.5% SDS, 50 mM EDTA). Single replicating DNA was detected with rat anti-CldU (Novus), mouse anti-IdU (Becton Dickinson) and anti-ssDNA (EMD Millipore) antibodies. Images were captured using the Nikon Eclipse TiE microscope and processed using NIS-Elements AR imaging software. BrdU incorporation and immunofluorescence To detect replication recovery, cells were pretreated with 3 μM APH for the indicated times and then incubated with 50 μM BrdU immediately for 15 min. After rinsing with phosphate-buffered saline (PBS), BrdU-labelled cells were fixed with 4% paraformaldehyde for 10 min. Cells were then permeabilized with 0.1% Triton X-100 in PBS for 2 min, denatured with 1.5 N HCl for 30 min. After PBS wash, cells were stained with mouse anti-BrdU antibody (BD Pharmingen) or in combination with rabbit anti-Rad51 antibody (Santa Cruz) and then with Alexa Fluor-conjugated secondary antibodies (Invitrogen). Images were captured using the Nikon Eclipse TiE microscope at a constant exposure time and data were quantitated with NIS Elements AR imaging software. iPOND analysis iPOND was performed largely as previously described [33] with the following modifications. Logarithmically growing cells ( ∼ 10 8 cells) were labelled with 10 μM EdU for 15 min, followed by HU treatment (2 mM, 2 h) to induce stalled forks. Cells, collected in 50 ml tubes, were washed three times with ice-cold PBS and transferred to 1.5 ml tubes. Cells were suspended with ice-cold nuclei extraction buffer (10 mM HEPES, 10 mM KCl, 1.5 mM MgCl2, 10% glycerol, 1 mM dithiothreitol, 0.34 M sucrose and 0.1% Triton X-100) containing protease inhibitors and incubated for 5 min at 4 °C. This buffer solubilizes the cytoplasm and keeps the nucleus intact. Cytoplasmic proteins were removed after centrifugation (400 × g , 5 min) at 4 °C. Nuclei were split evenly into two 1.5 ml tubes, one for the ‘click’ reactions to conjugate biotin to the EdU-labelled DNA and the other as the negative control by replacing biotin azide with dimethylsulphoxide for mock click reaction. Briefly, the nuclei pellets were resuspended with ice-cold click reaction mix (a 5 ml click reaction mix is sufficient for ∼ 5 × 10 7 cells) and incubated with rotation at 4 °C for 1 h. The samples were centrifuged for 10 min (400 × g , 4 °C) and the pellets were washed once with ice-cold PBS. Ice-cold lysis buffer (1% SDS in 50 mM pH8.0 Tris, 400 μl) with protease inhibitor was added to each sample for sonication, followed by centrifugation at the maximum speed for 10 min at 4 °C. The supernatants were diluted with 400 μl PBS to a total volume of 800 μl, 40 μl of which was used as input samples. Streptavidin beads were then used to capture the biotin-conjugated DNA-protein complexes overnight at 4 °C. Purified replication fork proteins were eluted by boiling in SDS-sample buffer, one-sixth of which was subjected to western blotting analysis. Cellular fractionation and western blotting For cellular fractionation, the ‘cytoplasmic soluble fraction’ was isolated by collection of the supernatant following centrifugation after incubation of cells in buffer A (10 mM HEPES at pH 7.9, 10 mM KCl, 1.5 mM MgCl 2 , 0.34 M sucrose and 10% glycerol) supplemented with protease inhibitors and 0.1% Triton X-100. Then the ‘nuclear-insoluble fraction’ was isolated by resuspending the pellets in buffer B (3 mM EDTA, 0.2 mM EGTA) supplemented with protease inhibitors for 30 min on ice followed by centrifugation. The supernatant was collected as the nuclear-soluble fraction, and pellets were collected as the nuclear-insoluble fraction. All samples were then subjected to western blotting. How to cite this article: He, J. et al. PTEN regulates DNA replication progression and stalled fork recovery. Nat. Commun. 6:7620 doi: 10.1038/ncomms8620 (2015).